Ultrathin high-temperature oxidation-resistant coatings of hexagonal boron nitride Hexagonal boron nitride is a two-dimensional layered material that can be stable at 1,500 °C in air and will not react with most chemicals. Here we demonstrate large-scale, ultrathin, oxidation-resistant coatings of high-quality hexagonal boron nitride layers with controlled thicknesses from double layers to bulk. We show that such ultrathin hexagonal boron nitride films are impervious to oxygen diffusion even at high temperatures and can serve as high-performance oxidation-resistant coatings for nickel up to 1,100 °C in oxidizing atmospheres. Furthermore, graphene layers coated with a few hexagonal boron nitride layers are also protected at similarly high temperatures. These hexagonal boron nitride atomic layer coatings, which can be synthesized via scalable chemical vapour deposition method down to only two layers, could be the thinnest coating ever shown to withstand such extreme environments and find applications as chemically stable high-temperature coatings. Recently, monolayers of hexagonal boron nitride (h-BN) have been successfully used as a smooth substrate for high-performance graphene devices [1] , [2] , [3] , [4] , [5] and as barrier materials in vertical heterostructures in combination with graphene and transition metal dichalcogenides [5] , [6] , [7] . Owing to the exceptional thermal and chemical stabilities [8] , h-BN could become an ideal coating material against oxidation at high temperatures if large area, high-quality, uniform atomic layers could be prepared on surfaces to be protected. Coating BN films on various surfaces such as two-dimensional (2D) layers and metals will considerably enhance the thermal and chemical stabilities of the materials. Traditionally, h-BN films have been prepared by pulsed laser deposition [9] ; however, this method will lead to amorphous BN films and have a relatively high cost. Mechanical exfoliation is an alternative approach to fabricate high-quality h-BN films but small h-BN footprints (typically, less than a few microns) limits its application as a coating. An easy and low-cost method is urgently needed for the h-BN films as a high-performance coating. In addition, integration of h-BN with other 2D materials such as graphene and transition metal dichalcogenides may considerately improve their working temperature and enhance the thermal dissipation. Bulk h-BN crystals have been synthesized using a high-temperature and high-pressure process for applications as far ultraviolet emitters [10] , [11] . However, the synthesis of atomically thin h-BN layers [12] , [13] , [14] , [15] has traditionally suffered from poor crystallization, making them inferior to flakes exfoliated from bulk samples resulting in relatively low performance [16] . In our previous work [12] , [13] , atomic layers of h-BN were synthesized on copper and nickel foils through low-pressure chemical vapour deposition (CVD) with ammonia borane as a precursor. Herein, we demonstrate that large-area and highly crystalline h-BN atomic layers can be synthesized via CVD method on Ni foil substrates and possess exceptional oxidation resistance for metals and other 2D layers such as graphene. Our method relies on sublimation of ammonia borane at 40~90 °C that is carried into the reaction region by Ar/H 2 gas flow, allowing a thickness-controlled formation of uniform h-BN films down to bilayers (see Supplementary Table S1 ). The copper and nickel foils are used for the substrates, because there are only small lattice mismatch between them and h-BN [17] . For other substrates such as Rh(111), h-BN mesh is observed due to the lattice mismatch [18] . The good quality of CVD-grown h-BN films are confirmed by complementary imaging and spectroscopic technologies such as optical imaging, scanning electronic microscopy (SEM), transmission electron microscopy (TEM), atomic force microscopy (AFM), Raman spectroscopy and X-ray photoelectron spectroscopy (XPS). Our experiments show that these ultrathin h-BN layers can be used as high-performance coatings to resist oxidation up to temperatures of up to 1,100 °C. The oxidation dynamic have been studied for h-BN-coated Ni via XPS depth profile. The weight gain and stoichiometry analysis of Ni oxides are analysed. In addition to metals surfaces, h-BN can also be coated on other 2D crystals such as graphene. We demonstrate graphene can be survived under 1,000 °C in air after oxidation for 2 min. The h-BN atomic coatings, on metals and graphene, could be the thinnest ever demonstrated coatings shown to withstand such extreme environments and could find important applications as chemically stable high-temperature coatings. Optical microscopy and TEM characterizations Optical evidence for h-BN growth on Ni foils is shown in Fig. 1a . It is shown that the dimensions of the h-BN layers grown can be up to 3 × 3 cm. The h-BN films can be transferred onto SiO 2 /Si substrates via a Poly(methyl methacrylate) (PMMA)-assisted method similar to that reported for graphene layer transfer [19] , as shown in Fig. 1b–d . The layer numbers from left to right are ~10, 5–6 and 2–3, respectively. A thick h-BN film on SiO 2 appears optically blue. Thinner layers produce a purple tint with decreasing brightness identified in a previous report [20] . The thickness and topography of the films are shown in the Supplementary Fig. S1 , showing that the films obtained are relatively smooth. More detailed characterization has been carried out using TEM and a scanning TEM (STEM) to assess the structure, crystallinity and the elemental content of the as-grown h-BN atomic layers. By controlling the growth temperature, growth time and precursor temperature, we are able to synthesize h-BN from double layers to several layers, as shown in Fig. 1e–h and Supplementary Table S1 . 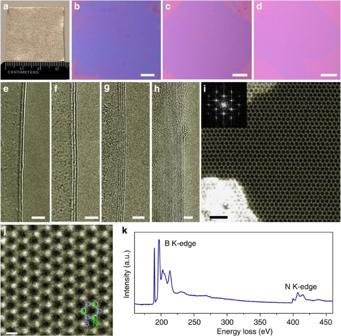Figure 1: Optical and TEM characterizations of CVD h-BN layers. (a) A photo of as-grown h-BN on Ni foils (size: ~3.5 × 3.5 cm2). (b–d) Optical image of bulk, few-layer (4~6) and double-layer h-BN films, respectively. Scale bars, 2 mm. (e–h) TEM images of double-, three-, four- and several-layered h-BN, respectively. Scale bar, 2 nm. (i) STEM–ADF image showing double-layered h-BN with AB stacking and its Fast Fourier Transform pattern (inset). Scale bar, 1 nm. (j) STEM–ADF image of single-layered h-BN after peeling off the bottom layer h-BN by electron beam. The brighter atoms are nitrogen and lighter ones are boron, as illustrated in the inset. Scale bar, 0.2 nm. (k) Electron energy loss spectrum of double-layered h-BN. Figure 1: Optical and TEM characterizations of CVD h-BN layers. ( a ) A photo of as-grown h-BN on Ni foils (size: ~3.5 × 3.5 cm 2 ). ( b – d ) Optical image of bulk, few-layer (4~6) and double-layer h-BN films, respectively. Scale bars, 2 mm. ( e – h ) TEM images of double-, three-, four- and several-layered h-BN, respectively. Scale bar, 2 nm. ( i ) STEM–ADF image showing double-layered h-BN with AB stacking and its Fast Fourier Transform pattern (inset). Scale bar, 1 nm. ( j ) STEM–ADF image of single-layered h-BN after peeling off the bottom layer h-BN by electron beam. The brighter atoms are nitrogen and lighter ones are boron, as illustrated in the inset. Scale bar, 0.2 nm. ( k ) Electron energy loss spectrum of double-layered h-BN. Full size image The interlayer spacing of few-layered h-BN is comparable to the lattice constant ~3.3 Å of bulk h-BN and to the estimates from theoretical calculations [21] . Because of the insulating nature and the susceptibility to radiation damage of few-layered h-BN films, a STEM working at 60 keV was employed for atomic structure evaluation and chemical analysis of the h-BN layers. Regions of defect-free h-BN layers were found and studied by STEM annular dark-field (ADF) imaging using the atomic number ( Z ) contrast. Most of the double-layered h-BN films were found to have AB stacking (Bernal stacking), which, along with AA’ stacking, is an energetically favourable structure according to ab initio calculations [21] . Relative rotations between layers were occasionally observed in few-layered h-BN ( Supplementary Fig. S2 ). Figure 1i presents a typical double-layered h-BN with AB stacking, where all of the atomic positions in the hexagonal rings display similar contrast due to the overlapping of B and N atoms from the two atomic layers. The inset is the corresponding Fast Fourier Transform pattern of the ADF image showing only one set of six-fold symmetric diffraction spots. When the bottom h-BN layer is peeled off by the electron beam, the atomic positions of B and N atoms in the monolayer h-BN can be directly identified via their ADF image intensities with N atoms being slightly brighter than B, as shown in Fig. 1j . Moreover, under our experimental conditions the ADF image intensity shows a quantized change as a function of numbers of h-BN layers ( Supplementary Fig. S2 ), which can be used to directly quantify the thickness of the h-BN samples. The size of single-crystal h-BN domains ranges from hundreds of nanometres to a few microns. The electron energy loss spectrum is acquired from a defect-free area of double-layered h-BN ( Fig. 1k ) showing both the boron K-edge (~190 eV) and nitrogen K-edge (~401 eV) features. The XPS, Raman and ultraviolet-absorption spectra of h-BN atomic layer can be found [17] in the Supplementary Figs S3–S5 . High-performance oxidation resistance coatings An immediate application of the grown h-BN atomic layers is their use as oxidation-resistant coatings of the underlying Ni surfaces in oxygen-rich environments at high temperatures. We performed oxidation experiments on Ni samples with and without h-BN atomic layer coating for 30 min at 1,100 °C in 300 mTorr oxygen. The Ni foils have been annealed before the oxidation experiments. The morphologies of the oxidized Ni foils were characterized by SEM microscopy. For the case where there was no h-BN coating, large number of oxide particles were formed on the Ni surface ( Fig. 2a,b ). Inset in Fig. 2b shows Ni oxide particles observed everywhere at the surfaces. With h-BN coatings, the nickel surface remained smooth and clean, and nickel grains were clearly observed ( Fig. 2c,d ). The parallel lines in Fig. 2c were produced during the polishing process of Ni foils. The thickness of the h-BN coating used was ~5 nm, as confirmed by AFM imaging ( Supplementary Fig. S6 ). Such ultrathin h-BN dielectric layer will significantly reduce the charging effect, which results to a clear secondary electron imaging [22] . We also transferred the 5-nm h-BN films to other metals, such as Cu and stainless steel, and confirmed the great performance of h-BN as oxidation-resistance coatings after PMMA-assisted transfer process ( Supplementary Fig. S6 ). We showed the h-BN coatings can also protect the surfaces of Cu and stainless steel films at 500 °C and 1,100 °C, respectively, for 30 min ( Fig. 2e–h ). It seems that sample transfer-induced topographical defects (such as cracks and pinholes) can be significantly reduced for 5 nm h-BN films. 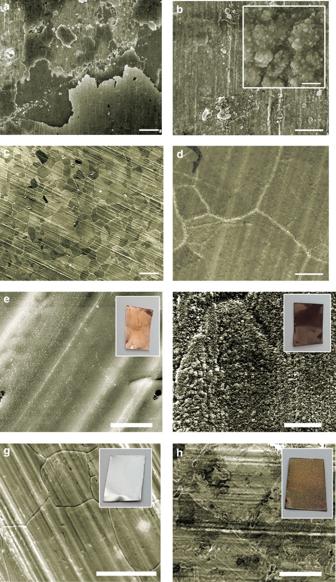Figure 2: h-BN thin films as high-performance oxidation-resistance coatings. (a,b) SEM images of pure Ni foils after oxidization at the same conditions. Ni oxide particles were formed on the surface. Scale bars, 100 μm (a), 10 μm (b) and 1 μm (binset). (c,d) SEM images of the 5 nm h-BN-coated Ni foils after oxidization in 300 mTorr oxygen at 1,100 °C for 30 min. The Ni oxides are clearly seen in the inset ofb, whereas Ni grains are found through the transparent h-BN films. Scales bars, 100 μm (c) and 10 μm (d). (e,f) SEM images of Cu foils after oxidization with and without h-BN coatings at 500 °C for 30 min. Scale bars, 5 μm (e,f). (g,h) SEM images of stainless steel surface with and without h-BN coatings at up to 1,100 °C for 30 min. The straight lines ineand g are from polish process. Scale bars, 40 μm (g,h). Insets ine–h: photos of each sample. With h-BN coating, both Cu and stainless steel can maintain their original colour. Without h-BN coatings, their colours have changed because of oxidation. Figure 2: h-BN thin films as high-performance oxidation-resistance coatings. ( a , b ) SEM images of pure Ni foils after oxidization at the same conditions. Ni oxide particles were formed on the surface. Scale bars, 100 μm ( a ), 10 μm ( b ) and 1 μm ( b inset). ( c , d ) SEM images of the 5 nm h-BN-coated Ni foils after oxidization in 300 mTorr oxygen at 1,100 °C for 30 min. The Ni oxides are clearly seen in the inset of b , whereas Ni grains are found through the transparent h-BN films. Scales bars, 100 μm ( c ) and 10 μm ( d ). ( e , f ) SEM images of Cu foils after oxidization with and without h-BN coatings at 500 °C for 30 min. Scale bars, 5 μm ( e , f ). ( g , h ) SEM images of stainless steel surface with and without h-BN coatings at up to 1,100 °C for 30 min. The straight lines in e and g are from polish process. Scale bars, 40 μm ( g , h ). Insets in e – h : photos of each sample. With h-BN coating, both Cu and stainless steel can maintain their original colour. Without h-BN coatings, their colours have changed because of oxidation. Full size image To carefully examine the oxidation resistance of the h-BN-coated Ni, XPS depth profiles were used to map the vertical out-of-plane elemental distribution across the coating/metal interface. A high-energy Ar ion beam accelerated by a voltage of 3 keV was used to etch the samples from its top surface, layer by layer, within a 2 × 2 mm area, as illustrated in Fig. 3a . The intensity evolution during etching is shown in Fig. 3b–d , for Ni, N and B, respectively. As the h-BN coating is very thin, a weak nickel signal could be collected even before Ar ion sputtering. For Ni, the main peak is located at ~852.6 eV. With sputtering, X-ray probes deeper into the sample and the intensity of Ni saturates after 15 s. For boron and nitrogen, their intensities decrease progressively to zero during sputtering. The peak of nitrogen is at ~398.2 eV, very close to the reported position of the N 1-s spectrum (398.1 eV) [23] , [24] , [25] . The most prominent peak for boron is ~190.9 eV, identical to hexagonal phase boron nitride [23] , [24] , [25] . It is noted that following the Ar-ion etching, the peak of B 1-s shifts from ~191 (h-BN) to ~188 eV (ref. 26 ), possible evidence showing that boron may be dissolved in Ni surface at high temperature. 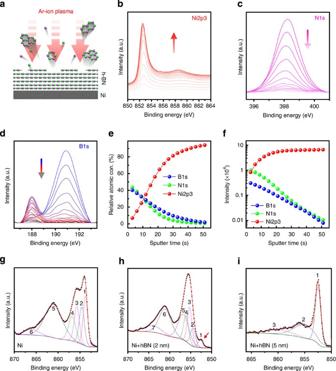Figure 3: XPS characterizations of h-BN-coated Ni foils. (a) Schematic shows the etching process of h-BN-coated Ni foil. (b–d) The XPS spectra of Ni (2p3), N (1 s) and B (1 s), respectively, acquired after each etching. The arrows indicate the evolution of the spectra. (e–f) Relative atomic concentration and intensity of each element versus sputtering time. (g–i) Individual Ni XPS spectra of pure Ni, 2 nm h-BN-coated Ni and 5 nm h-BN-coated Ni foils after oxidation testing. Figure 3: XPS characterizations of h-BN-coated Ni foils. ( a ) Schematic shows the etching process of h-BN-coated Ni foil. ( b – d ) The XPS spectra of Ni (2p3), N (1 s) and B (1 s), respectively, acquired after each etching. The arrows indicate the evolution of the spectra. ( e – f ) Relative atomic concentration and intensity of each element versus sputtering time. ( g – i ) Individual Ni XPS spectra of pure Ni, 2 nm h-BN-coated Ni and 5 nm h-BN-coated Ni foils after oxidation testing. Full size image The evolutions of the atomic concentration and peak intensity of Ni, N and B as a function of sputtering time are plotted in Fig. 3e,f . The two plots show a similar trend, suggesting the formation of an effective h-BN protection layer over the Ni substrate. Figure 3g–i show the XPS spectra (Ni 2p) of post-oxidation pure Ni foil, and Ni foils with 2 and 5 nm h-BN coatings. For the pure Ni foil, high-temperature oxidation resulted in dominant peaks at ~853.7, 855.7 and 861.0 eV, corresponding to the main peaks of Ni oxides ( Supplementary Fig. S7 and Supplementary Table S2 ) [27] . With 2 nm h-BN coating, although prominent signals are found from Ni oxides, a weak peak at ~852.6 eV from pristine Ni, marked by the red arrow, appears ( Supplementary Fig. S8 and Supplementary Table S3 ). With 5 nm h-BN coating, the spectra evidently change from a typical Ni oxide profile to a pure Ni profile with a main peak located at ~852.5 eV and two well-known satellite peaks ( Supplementary Fig. S9 and Supplementary Table S4 ). These observations suggest that a high-quality h-BN coating with an appropriate thickness has a very good potential to significantly improve oxidation resistance of metals at high temperatures and under oxygen-rich atmospheres. To systematically study the oxidation protection offered by h-BN coatings, 2- and 5-nm h-BN films were deposited on Ni foils by the CVD method. We first oxidized all three samples (pristine Ni foil and Ni foil with 2 and 5 nm h-BN coating, respectively) in air at different temperatures ranging from 200 °C to 1,100 °C ( Fig. 4a ). The oxidation duration was kept the same at 5 min. With the presence of the h-BN coating, the net weight gain due to oxidation dropped from ~5.4% (for pristine Ni foils) to ~3.2% (for Ni foil with 2 nm h-BN coating), to ~1.5% (for Ni foil with 5 nm h-BN coating) after oxidation of the coated and uncoated foils in air at 1,100 °C. A parabolic behaviour of the oxidation kinetics was observed from 800 °C to 1,100 °C, as plotted in the inset of Fig. 4a , consistent with previous reports on oxidation kinetics [28] . Furthermore, the oxidation durations versus weight gain is presented in Fig. 4b , at 1,100 °C and under 300 mTorr oxygen atmosphere. The gained weight saturates after oxidation for 1 h and, again, 5 nm h-BN coating dramatically reduced this value by >70% compared with the pristine Ni foil (from 13.4% to 3.01%). At 1,100 °C, the oxidation follows the parabolic rate law (inset in Fig. 4b ). The oxidation depth of Ni foil versus time is plotted in false-coloured contours ( Fig. 4c,d ). The colour represents the stoichiometry of nickel oxides in atomic concentration ratio, derived from the XPS depth profile in a total time of 5 min with an interval of 1 min. Pure or slightly oxidized nickel regions are shown in blue, moderately oxidized nickel (Ni/O~1) is in green, while yellow and red refers to heavily and fully oxidized Ni (Ni 2 O 3 ), respectively. The white dotted-contour lines indicate the rough boundaries of NiO formed. As can be observed in the plot, with 5 nm h-BN coating the blue region dominates. A small red area is found on the surface of Ni foils. In sharp contrast, without the h-BN coating, green region dominates and the red region propagates deep into the Ni substrate. More than five locations have been etched at each temperature and result to similar oxidation profiles. 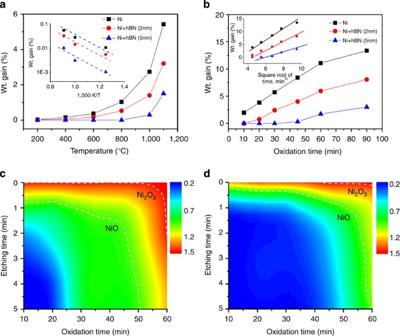Figure 4: Weight gain and stoichiometry analysis of Ni oxides. (a) Weight gain versus temperature of pristine Ni foils, 2- and 5 nm h-BN-coated Ni foils. Oxidation duration is 5 min in air. Inset shows the parabolic rate constant as a function of the inverse absolute temperature from 800 °C to 1,100 °C. (b) Weight gain versus oxidizing duration at 1,100 °C in 300 mT oxygen atmosphere. Inset represents the weight gain as a function of the square root of time. (c,d) Contours showing the depth profile of Ni oxidization profiles for durations from 10 to 60 min. The oxidations were performed at 1,100 °C and under 300 mT oxygen atmosphere. The colours indicate the oxidation level represented by the atomic concentration of oxygen over nickel from slight (blue) to heavy (yellow and red) oxidation. White dotted line is the contour lines indicating the boundaries of NiO. Figure 4: Weight gain and stoichiometry analysis of Ni oxides. ( a ) Weight gain versus temperature of pristine Ni foils, 2- and 5 nm h-BN-coated Ni foils. Oxidation duration is 5 min in air. Inset shows the parabolic rate constant as a function of the inverse absolute temperature from 800 °C to 1,100 °C. ( b ) Weight gain versus oxidizing duration at 1,100 °C in 300 mT oxygen atmosphere. Inset represents the weight gain as a function of the square root of time. ( c , d ) Contours showing the depth profile of Ni oxidization profiles for durations from 10 to 60 min. The oxidations were performed at 1,100 °C and under 300 mT oxygen atmosphere. The colours indicate the oxidation level represented by the atomic concentration of oxygen over nickel from slight (blue) to heavy (yellow and red) oxidation. White dotted line is the contour lines indicating the boundaries of NiO. Full size image Graphene is another material that can benefit from having an ultrathin h-BN coating, especially due to the structural similarities of both the materials. Recently, h-BN films have been considered complementary substrates of graphene devices [29] , [30] . Here we show that the graphene layers can survive elevated temperatures as high as 1,000 °C if a h-BN atomic layer is coated on top as an oxidation-resistant coating. Few-layered h-BN can be either transferred or directly grown on single-layered graphene on a 285 nm SiO 2 substrate ( Supplementary Figs S10–12 ) [13] . The h-BN-coated graphene can be found to locate in the top portion of Fig. 5a,b . The thickness of the h-BN coating is ~2 nm ( Supplementary Fig. S11 ). The underlying graphene layer is continuous and fully covers the SiO 2 substrate. However, at few locations graphene is broken and the SiO 2 can be seen underneath these broken regions, as indicated by the white arrow. The G/h-BN sample was then oxidized at 1,000 °C in air for 2 min. The typical morphology after oxidation is shown in Fig. 5b . It is observed that the uncovered graphene has been burned away and h-BN-covered graphene still survives. To systematically study the oxidation rate of h-BN-coated graphene, in-situ temperature-dependent Raman characterization ( Fig. 5c–f ) was carried out from room temperature to 1,000 °C for both pristine graphene and h-BN-covered graphene. At each temperature, Raman spectra were recorded at more than five different locations in each sample. The Raman signature dependence on temperature is represented in Fig. 5c,d in a false coloured contour. Below 500 °C, there are no obvious changes in the Raman spectra for both types of graphene samples. For pristine graphene samples, at a temperature above 500 °C, its D and D′ peaks appear while G and 2D peaks become weaker, suggesting that the oxidation has significantly degraded the graphene structure. There is no Raman peak observed in the bare graphene after oxidation above 700 °C. In contrast, for the h-BN-coated graphene the D and D′ peaks were not seen until oxidation above 800 °C. The sample could retain a good Raman signature for graphene materials even after oxidation at a temperature up to 1,000 °C, confirming the protective nature of the h-BN coatings. The Raman spectra at 200, 600 and 1,000 °C are shown in Fig. 5e,f . Finally, we test oxidation-resistant coating effect of h-BN for graphene on sapphire substrate. As shown in Supplementary Fig. S12 , a very good anti-oxidation performance has again been observed. 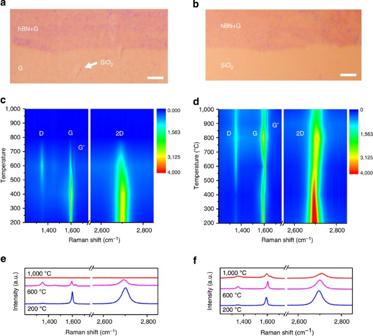Figure 5: h-BN films as an anti-oxidation layer for graphene. (a) Optical image of graphene coated by 2 nm h-BN layers on the silica substrate. Bottom region is pure graphene and top one is h-BN on graphene. Scale bar, 2 μm. (b) Optical image of h-BN-coated graphene after 2 min oxidation at 1,000 °C. Uncovered graphene (bottom) was burned out and h-BN-covered one still survived (top). Scale bar, 2 μm. (c,d) Contours of Raman spectra as a function of oxidation temperature acquired from (c) uncovered graphene and (d) h-BN-coated graphene (d) that have been oxidized under a controllable temperature. (e,f) Typical Raman spectra for the bare and h-BN-coated graphene, respectively, under 200, 600 and 1,000 °C. Figure 5: h-BN films as an anti-oxidation layer for graphene. ( a ) Optical image of graphene coated by 2 nm h-BN layers on the silica substrate. Bottom region is pure graphene and top one is h-BN on graphene. Scale bar, 2 μm. ( b ) Optical image of h-BN-coated graphene after 2 min oxidation at 1,000 °C. Uncovered graphene (bottom) was burned out and h-BN-covered one still survived (top). Scale bar, 2 μm. ( c , d ) Contours of Raman spectra as a function of oxidation temperature acquired from ( c ) uncovered graphene and ( d ) h-BN-coated graphene ( d ) that have been oxidized under a controllable temperature. ( e , f ) Typical Raman spectra for the bare and h-BN-coated graphene, respectively, under 200, 600 and 1,000 °C. Full size image We can gain insight to our experimental observations by considering the main high-temperature oxidation reaction of boron nitride with oxygen [31] : where the standard formation enthalpy of B 2 O 3 in its liquid phase is Δ H f =−1,253 KJ M −1 , or equivalently ~13 eV is released for every two B atoms that are oxidized. This reaction involves the removal of two pairs of BN molecules. The energy required to remove the B atoms from the structurally stable h-BN crystal is ~11.2 eV for one atom and about ~20 eV for the removal of two nearby B atoms [32] . As vacancy formation energies are drastically reduced when neighbouring atoms are removed sequentially, the average removal energy cost for two B atoms is expected to be ~15 eV when the oxidation of B is assisted by the removal of neighbouring N atoms during the reaction through the formation of N 2 or oxidized nitrogen in any of the NO X varieties. Despite the large barrier towards divacancy formation, the total reaction energy balance Δ H ~ H 2BN vac −9.8−13=−7.8 eV remains exothermic. In this estimate, we used the nitrogen molecule bond energy 9.8 eV and the somewhat low estimate value H 2BN vac ~15 eV for the average BN divacancy formation energy. The energy released in the removal and oxidation of two pairs of B and N atoms is therefore comparable in magnitude to the oxidation energy of two carbon atoms in graphite where, in each reaction, with the standard reaction enthalpy of Δ H f =−393 KJ M −1 releases ~4 eV per one removed carbon atom. Thus, the high temperature required for the oxidation of h-BN must be traced back to the large energy required in activating the reaction. In a graphene sheet, the initial vacancy formation energy is ~7.5 eV (ref. 33 ), whereas the removal of contiguous carbon sites can be done at negligible additional cost. This is substantially smaller than the ~15 eV required for the formation of the two BN divacancies needed in an elementary oxidation reaction. Therefore, the large activation barrier in h-BN in the free-energy landscape can be attributed to the large formation energies of the initial vacancies and to the fact that an elementary oxidation reaction in h-BN involves the simultaneous removal of more atoms than in graphene. These observations explain why the h-BN sheets start to oxidize at a much higher temperature than graphene. In conclusion, we have shown the excellent oxidation protection offered by atomically layered h-BN and its suitability as an ideal ultrathin coating material. The thicknesses of h-BN layers can be well controlled from double to few layers, and the size can be up to a few centimetres. The few-layer h-BN films can work as excellent passivation coatings at temperatures up to 1,100 °C in oxygen-rich atmospheres. The h-BN coatings we have developed here are the thinnest ever coatings that have been used at such high temperatures, remaining stable and protecting metal surfaces from high-temperature oxidation. These ultrathin coatings should find exciting applications as protective layers for thin metal films, graphene and transition metal dichalcogenides electronics in extreme conditions. Synthesis of h-BN atomic layers on Ni foils The synthesis of h-BN was carried out in a quartz tube furnace. A nickel foil with a thickness of 12.5 μm (Goodfellow, Inc., purity: 99.9%) was placed in the centre of the quartz tube furnace. The quartz tube was pumped down to 60 mT during growth. The temperature was raised to 1,000 °C in 50 min under the protection of 300 mTorr Ar/H 2 gas flow (15 vol% H 2 balanced by 85 vol% Ar), and subsequently ammonia borane (NH 3 –BH 3 ), as precursors, was sublimated at ~40–90 °C as the source of B and N. The typical growth time is about 1–2 h. The temperature of ammonia borane and the growth time are two main factors to control the thickness of h-BN film. The thicknesses of h-BN layers can be well controlled from double layer to more than ten layers with optimized growth conditions. The heating temperature of ammonia borane precursor and substrate (Ni foils) are crucial for controlling the thickness of h-BN films. The growth conditions are listed in Supplementary Table S1 . Double-layered h-BN can be synthesized under ~1,000 °C by heating precursor as low as 40 °C. The growth time is 1 h. A longer growth time results to a thicker h-BN film. As expected, higher precursor temperature and growing temperature will enhance the growth rate of h-BN. After growth, the furnace was cooled down to room temperature slowly. Afterwards, the Ni foils were coated with PMMA to transfer h-BN to other substrates for further characterizations. Characterizations of h-BN/Ni and h-BN/graphene structures AFM (Agilent PicoScan 5500 and Veeco Digital Instrument Nanoscope IIIA) was used to determine the thicknesses and roughness of the samples. XPS (PHI Quantera XPS) was performed using monochromatic aluminum Kα X-rays. Depth profiles were performed with a 3-keV Ar ion beam and alternative mode within an etching area of 0.5 mm × 0.5 mm to etch the h-BN-coated Ni foils. Raman spectroscopy (Renishaw inVia) was performed at 514.5 nm laser excitation at a power of 20 mW. Field-emission SEM (JEOL 6500F) was used to characterize the morphology of the Metal foils (Ni, Cu, stainless steel) with and without h-BN coatings after oxidations. High-resolution TEM (JEOL-2100) was employed to study the morphologies of h-BN layers at an accelerating voltage of 200 keV. The STEM experiments were performed on an aberration-corrected Nion UltraSTEM 100 operating at 60 keV (ref. 34 ). Electron energy loss spectra were collected using a Gatan Enfina spectrometer with 48 mrad collection semi-angle. The convergence semi-angle for the incident probe was 31 mrad, and ADF images were collected for a half-angle range of ~54–200 mrad. How to cite this article: Liu, Z. et al . Ultrathin high-temperature oxidation-resistant coatings of hexagonal boron nitride. Nat. Commun. 4:2541 doi: 10.1038/ncomms3541 (2013).